Australia’s arid-adapted butcherbirds experienced range expansions during Pleistocene glacial maxima A model of range expansions during glacial maxima (GM) for cold-adapted species is generally accepted for the Northern Hemisphere. Given that GM in Australia largely resulted in the expansion of arid zones, rather than glaciation, it could be expected that arid-adapted species might have had expanded ranges at GM, as cold-adapted species did in the Northern Hemisphere. For Australian biota, however, it remains paradigmatic that arid-adapted species contracted to refugia at GM. Here we use multilocus data and ecological niche models (ENMs) to test alternative GM models for butcherbirds. ENMs, mtDNA and estimates of nuclear introgression and past population sizes support a model of GM expansion in the arid-tolerant Grey Butcherbird that resulted in secondary contact with its close relative—the savanna-inhabiting Silver-backed Butcherbird—whose contemporary distribution is widely separated. Together, these data reject the universal use of a GM contraction model for Australia’s dry woodland and arid biota. Global cooling during Pleistocene glacial maxima (GM) is recognized as having had an important influence on the structure of current biodiversity [1] . The widely accepted GM contraction model of Pleistocene biogeography [1] grew from initial examples of temperate species in the Northern Hemisphere. These exhibited substantial range contractions and differentiation in one or few refugia during GM, followed by range expansions, secondary contact and gene flow during warmer interglacials (glacial minima). However, the GM contraction model is not universally applicable to biota from unglaciated regions such as those in Africa, Australia, South America and the Northern Hemisphere [2] , [3] , [4] , [5] , [6] , [7] , [8] , [9] , or cold-adapted taxa in the Northern Hemisphere [10] , [11] . Indeed, an inverse model of GM expansion has been proposed for cold-adapted taxa in the Northern Hemisphere [1] , [10] , wherein populations underwent range expansions and gene flow during GM, followed by range contractions to cooler higher latitudes or higher elevations during interglacials. The response of Australia’s arid-tolerant biota to increasing aridity during GM should be analogous to that of Northern Hemisphere cold-tolerant biota [1] , [10] . That is, arid-tolerant biota tracked the expansion of dry woodland, semi-arid and arid habitats during cooler and drier GM, and contracted during warmer and wetter interglacials, such as at present. This GM expansion model is supported by palaeoclimatic reconstructions ( Fig. 1 ) [7] , [8] , palaeo-ENMs from Northern Australia [12] , [13] and phylogeographic structure [14] , [15] , which suggest that many widespread arid-tolerant taxa could have maintained large populations throughout the Pleistocene as a result of the long-term availability of suitable arid habitats [7] . However, despite this evidence, the dominant assumption in the literature relating to Australian biota remains one of range contraction and population persistence in refugia during GM [14] , [15] . Given an assumption of GM contraction, the lack of congruence among phylogeographic patterns and evidence for large population sizes through time in many species have been attributed to populations persisting in multiple, ‘idiosyncratic’ (species-specific), GM refugia that were dispersed across the continent [14] , [16] rather than the few, mostly coastal, GM refugia hypothesized for Australia’s mesic-adapted biota [17] . These dispersed GM refugia are functionally similar to the ‘cryptic refugia’ and ‘pockets of favourable microclimates’ invoked for New Zealand temperate trees and some taxa in central Europe [5] , [18] , [19] , [20] , [21] . However, these implicitly involve reductions in population size, while Australian examples are invoked to explain the maintenance of large population sizes throughout the Pleistocene [14] . 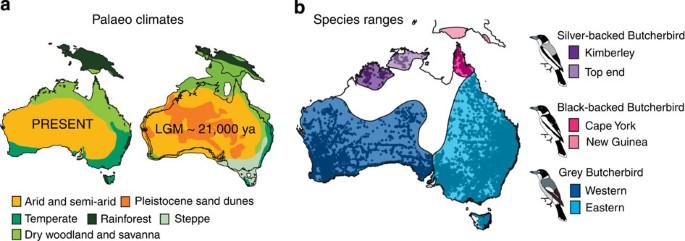Figure 1: Expansion of dry habitats inhabited by white-throated butcherbirds during the last glacial maximum. (a) Major habitat types in Australia and New Guinea at present (data from Schodde68) and during the LGM (data from Hopeet al.8) when sea levels were lower, the arid zone expanded and extensive sand-dunes were active. The approximate extent of Pleistocene sand-dunes is shown in dark orange (data from Williamset al.69and Byrneet al.14). (b) Geographic range of white-throated butcherbirds (data from Schodde and Mason22) overlays occurrence records for each species from the Birds Australia Birdata Project (www.birdata.com.au) and the Australian National Wildlife Collection. Cartoons show the major plumage differences between the three species: (i) back colour, (ii) presence or absence of white lores (eye-spots), (iii) presence or absence of black chin spot, (iv) pure-white versus off-white/grey ventrum and (v) amount of white on wing. The range of each species is divided into two geographic groups that correspond to phenotypically or genetically differentiated forms that are often treated as subspecies (Kimberley:C. a. argenteus; Top End:C. a. colletti; New Guinea:C. m. mentalis; Cape York:C. m. kempi; western Grey:C. t. leucopterus sens. strict.; eastern Grey:C. t. colei,C. t. torquatus, C. t. cinereus22). Figure reproduced with permission from Elsevier23. Figure 1: Expansion of dry habitats inhabited by white-throated butcherbirds during the last glacial maximum. ( a ) Major habitat types in Australia and New Guinea at present (data from Schodde [68] ) and during the LGM (data from Hope et al. [8] ) when sea levels were lower, the arid zone expanded and extensive sand-dunes were active. The approximate extent of Pleistocene sand-dunes is shown in dark orange (data from Williams et al. [69] and Byrne et al. [14] ). ( b ) Geographic range of white-throated butcherbirds (data from Schodde and Mason [22] ) overlays occurrence records for each species from the Birds Australia Birdata Project ( www.birdata.com.au ) and the Australian National Wildlife Collection. Cartoons show the major plumage differences between the three species: (i) back colour, (ii) presence or absence of white lores (eye-spots), (iii) presence or absence of black chin spot, (iv) pure-white versus off-white/grey ventrum and (v) amount of white on wing. The range of each species is divided into two geographic groups that correspond to phenotypically or genetically differentiated forms that are often treated as subspecies (Kimberley: C. a. argenteus ; Top End: C. a. colletti ; New Guinea: C. m. mentalis ; Cape York: C. m. kempi ; western Grey: C. t. leucopterus sens. strict. ; eastern Grey: C. t. colei , C. t. torquatus, C. t. cinereus [22] ). Figure reproduced with permission from Elsevier [23] . Full size image Our goal is to evaluate GM expansion–contraction models for Australia’s arid-tolerant biota using the white-throated butcherbird group (Artamidae, Cracticus subgenus Bulestes ). This group comprises three species that together occur across most of Australia’s woodland, semi-arid and arid habitats ( Fig. 1 ). The Grey Butcherbird ( C. torquatus ) is found across southern Australia in temperate, dry, semi-arid and arid woodland habitats but is absent from the deserts of central Australia and the monsoon tropics of northern Australia. The Silver-backed Butcherbird ( C. argenteus ) occurs in the drier savanna habitats of monsoonal northwestern Australia. The Black-backed Butcherbird ( C. mentalis ) occurs in the higher rainfall savanna habitats of northeastern Australia and southern New Guinea. The three species are currently geographically isolated from each other—Silver-backed and Grey, in particular, by at least 900 km of arid and savanna habitat and large tracts of sand-dune dominated deserts—and have distinctive plumage traits that differentiate the species boundaries [22] . However, none are reciprocally monophyletic with respect to another at either mtDNA or nuclear loci [23] . The pattern of mtDNA paraphyly [23] is best explained by a historical range expansion that resulted in secondary contact and introgression of either Grey or Black-backed Butcherbirds into Silver-backed Butcherbirds. However, this pattern could also originate from incomplete lineage sorting or incorrect taxonomy. We propose that, for a species response to fit a GM contraction model, the species must have undergone a substantial reduction in range and population size (that is, a demographic bottleneck) compared with the current interglacial. This interpretation follows the dominant assumption in the literature that GM climates were less suitable for arid-tolerant biota than at present, and thus caused species to retreat to, and persist in, refugia. However, we emphasize that, if the GM range or population size of a species is greater than, equal to or only slightly reduced compared with interglacials, then this species response cannot be viewed as a contraction to a refuge. In contrast, a substantial range and population size expansion at GM compared with the current interglacial would fit a GM expansion model, while little or no change in range or population size would fit either a GM range stability or range shift model depending on whether the range of the species underwent a latitudinal shift [5] . To assess alternative GM models we use ecological niche modelling (ENM) under the current interglacial and the last glacial maximum (LGM: 18–23 kya), and multilocus coalescent analyses. Under a GM expansion model, there should be (1) coalescent evidence for introgression of either Grey or Black-backed Butcherbirds into Silver-backed Butcherbirds, (2) ENM predictions of range expansion and secondary contact at LGM and (3) coalescent evidence of demographic expansions that are congruent with ENMs. Species-ecology and palaeoclimatic reconstructions predict two GM expansion scenarios that involve either secondary contact following an expansion of Grey Butcherbirds into the Silver-backed Butcherbird range as they tracked expanding dry habitats, or secondary contact following a northward range shift on the exposed Arafura shelf in either, or both, Silver-backed and Black-backed Butcherbirds as they tracked savanna habitats ( Fig. 1 ). Under a GM contraction model, there should be (1) no coalescent evidence of introgression (that is, mtDNA paraphyly results from incomplete lineage sorting or incorrect taxonomy), (2) ENM predictions of range contraction at LGM (whether to multiple dispersed refugia sensu Byrne et al. [14] or large stable refugia sensu Keast [24] ) and (3) coalescent evidence of demographic bottlenecks that are congruent with ENMs. We find that all lines of evidence support a model of GM expansion for the arid-tolerant Grey Butcherbird. Specifically, eastern populations of the Grey Butcherbird underwent range expansion, resulting in nuclear and mitochondrial introgression with the Silver-backed Butcherbird in northwestern Australia. These findings go against the current paradigm for Australian fauna of universal GM contraction to refugia, and we call for careful testing of alternative GM models across co-distributed taxa. Phylogeography This study expands on the systematic study of Kearns et al. [23] by adding 54 individuals to the mtDNA ND2 data set and three nuclear introns ( ACTB-3, FN1-31 and RPL37A-3 ) to the four introns previously sequenced ( BF-7, BRM-15, GAPDH-11 and ODC-6 & 7 ). Bayesian phylogenetic analysis of 138 white-throated butcherbird mitochondrial, ND2 , sequences provided strong support (posterior probability >0.9) for two divergent clades (uncorrected P distance: 4.8%; Dxy : 4.3%; see Supplementary Table 1 ) ( Fig. 2 ; Supplementary Fig. 1 ). Of the 36 Silver-backed Butcherbirds sequenced for ND2 , 23 were grouped into Clade 1 with Grey Butcherbirds ( n =86) and 13 were grouped into Clade 2 with Black-backed Butcherbirds ( n =13; Fig. 2 ). Unrooted parsimony networks and measures of net-sequence divergence ( Dxy ) showed that Clade 1 Silver-backed Butcherbird haplotypes were more closely related to those of eastern Grey Butcherbirds ( Dxy : 1.0%) than those of eastern and western Grey Butcherbirds are to each other ( Dxy : 1.9%), and than Clade 2 Silver-backed Butcherbird haplotypes are to those of Black-backed Butcherbirds ( Dxy : 1.7%). 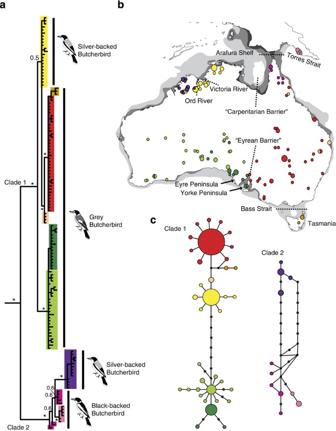Figure 2: Phylogeographic structure of paraphyletic mtDNA lineages. (a) Bayesian inference places mitochondrialND2haplotypes from Silver-backed Butcherbirds in two deeply divergent clades (Dxy=4.34%; uncorrectedPdistance=4.8%) that are grouped with either Grey Butcherbirds (Clade 1) or Black-backed Butcherbirds (Clade 2). Colours indicate nine major haplotype groups. Asterisks indicate key nodes with >0.90 posterior probability. Numbers above branches indicate posterior probability values for key nodes with <0.9 posterior probability. (b) Geographic structuring of mtDNA haplotype groups. Contours on the map show extent of land exposed at various times in the Pleistocene (10 m (dark grey), 40 m (medium grey) and 120 m (light grey) below present—data from Voris70). (c) Unrooted network ofND2haplotypes. Black circles in the haplotype networks represent inferred, but unsampled, haplotypes. In both the map and the haplotype networks the size of the circles are proportional to sampling frequency. Analysis of molecular variance indicated that mtDNA was differentiated across species boundaries despite the lack of reciprocal monophyly ( F st 0.59, P <0.0001; Supplementary Table 2 ). MtDNA also showed strong geographic structuring across barriers to dispersal that have been previously postulated for other butcherbirds [25] , [26] , [27] and other arid-tolerant biota [14] , [15] (for example, Eyrean Barrier, Carpentarian Barrier, Ord and Victoria River arid intrusions; Fig. 2 ; Supplementary Table 2 ). Notably, Clade 2 Silver-backed haplotypes are restricted to west of the Ord River arid intrusion in the Kimberley ( sensu Ford [28] ), whereas Clade 1 Silver-backed haplotypes are restricted to east of the Ord River with the exception of five individuals ( Fig. 2 ). One BRM-15 allele was restricted to populations west of the Victoria River in the Kimberley ( Fig. 3 ). ODC-6 & 7 and GAPDH-11 each had an allele found only in Silver-backed Butcherbirds that was almost exclusively sampled in individuals from the Kimberley ( Fig. 3 ). Figure 2: Phylogeographic structure of paraphyletic mtDNA lineages. ( a ) Bayesian inference places mitochondrial ND2 haplotypes from Silver-backed Butcherbirds in two deeply divergent clades ( Dxy =4.34%; uncorrected P distance=4.8%) that are grouped with either Grey Butcherbirds (Clade 1) or Black-backed Butcherbirds (Clade 2). Colours indicate nine major haplotype groups. Asterisks indicate key nodes with >0.90 posterior probability. Numbers above branches indicate posterior probability values for key nodes with <0.9 posterior probability. ( b ) Geographic structuring of mtDNA haplotype groups. Contours on the map show extent of land exposed at various times in the Pleistocene (10 m (dark grey), 40 m (medium grey) and 120 m (light grey) below present—data from Voris [70] ). ( c ) Unrooted network of ND2 haplotypes. Black circles in the haplotype networks represent inferred, but unsampled, haplotypes. In both the map and the haplotype networks the size of the circles are proportional to sampling frequency. 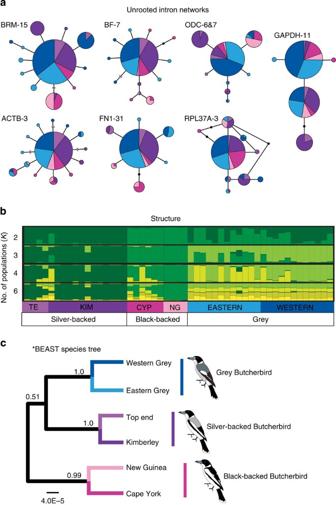Figure 3: Test of species boundaries using nuclear loci. (a) Phased allele networks for seven nuclear loci scaled by sample size, and coloured according to the six geographic groups used asa prioritaxonomic units in *BEAST. Small black circles represent inferred unsampled haplotypes, and white boxes indicate the positions of indels. (b) STRUCTURE plots depicting population assignment of 51 white-throated butcherbirds estimated under two, three, four and six putative populations (K). Each vertical bar represents the proportion of assignment of a single indivual to each population considered at that value ofK. Individuals are sorted by geographic group and species—Top End (TE), Kimberley (KIM), Cape York (CYP), New Guinea (NG), eastern Grey Butcherbird (EASTERN), western Grey Butcherbird (WESTERN). (c) *BEAST multilocus species tree supporting the monophyly of the three white-throated butcherbird species. Figure reproduced with permission from Elsevier23. Full size image Figure 3: Test of species boundaries using nuclear loci. ( a ) Phased allele networks for seven nuclear loci scaled by sample size, and coloured according to the six geographic groups used as a priori taxonomic units in *BEAST. Small black circles represent inferred unsampled haplotypes, and white boxes indicate the positions of indels. ( b ) STRUCTURE plots depicting population assignment of 51 white-throated butcherbirds estimated under two, three, four and six putative populations ( K ). Each vertical bar represents the proportion of assignment of a single indivual to each population considered at that value of K . Individuals are sorted by geographic group and species—Top End (TE), Kimberley (KIM), Cape York (CYP), New Guinea (NG), eastern Grey Butcherbird (EASTERN), western Grey Butcherbird (WESTERN). ( c ) *BEAST multilocus species tree supporting the monophyly of the three white-throated butcherbird species. Figure reproduced with permission from Elsevier [23] . Full size image Tests of species boundaries using nuclear loci To assess whether the mtDNA phylogeny accurately reflected the speciation history of white-throated butcherbirds, we used seven nuclear introns to delimit species boundaries and estimate a multilocus species tree. Each locus showed low to moderate structuring by species ( Supplementary Table 2 : F st 0.05–0.43, P <0.01) despite extensive sharing of alleles among species ( Fig. 3 ). Two approaches were used to delimit species boundaries: (1) multispecies coalescent species tree algorithm in *BEAST [29] using the six major geographic groups indicated by mtDNA and subspecies as a priori ‘species boundaries’ (that is, western and eastern Grey Butcherbirds, Top End and Kimberley Silver-backed Butcherbirds, New Guinea and Cape York Black-backed Butcherbirds; Figs 1 and 2 ) and (2) Bayesian clustering algorithm in STRUCTURE [30] that determines the number of genetic groups without a priori information about species boundaries. The *BEAST species tree strongly supports the monophyly of each of the three species (posterior probability >0.99); however, there was no well-supported relationship among them ( Fig. 3 ). STRUCTURE analyses using a subset of 51 individuals sampled for all seven nuclear loci were broadly consistent with morphology-based species boundaries ( Fig. 3 ). Log-likelihoods peaked at K =3 and then plateaued, remaining similar up to K =8. The three genetic clusters identified at K= 3 corresponded to the three species. However, the delta K method supported K =4 as the best-fit number of genetic clusters for the data set ( Fig. 3 ). The assignment of nine Grey, one Silver-backed and one Black-backed individuals to a fourth genetic cluster could be the result of gene flow. Tests for nuclear introgression Owing to uncertainty in relationships of the three species of Butcherbirds ( Fig. 3 ), demographic parameters (divergence time ( t ), effective population size ( Ne ) and population migration rate ( 2NM )) were estimated in the Isolation with Migration (IMa2) [31] programme for two different three-population models that reflected the two plausible species trees indicated by the mtDNA phylogeny ( Fig. 2 )—Tree 1: where Silver-backed and Black-backed are sisters, and Tree 2: where Silver-backed and Grey are sisters. IMa2 estimates for these two alternative species trees overlapped substantially and neither analysis had closed posterior densities for the divergence time parameters ( t ), and the upper bound of both t 1 and t 0 had to be constrained in order to obtain adequate mixing and convergence ( Supplementary Fig. 2 ; Supplementary Table 3 ). In both analyses, posterior probabilities for t 1 and t 0 were highest within the past one million years, and 95% highest posterior density credibility intervals encompassed a broad range of dates (~3,000–5,821,000 ya; Supplementary Table 3 and Supplementary Fig. 2 ). Effective population size estimates were largest for Grey (~57,000–396,000) and similar for Black-backed (~6,000–147,000) and Silver-backed (~3,000–88,000) Butcherbirds ( Supplementary Table 3 ; Supplementary Fig. 2 ). Irrespective of the species tree used, an assumption of no nuclear introgression ( m =0) was rejected for both Grey into Silver-backed Butcherbirds and Grey into Black-backed Butcherbirds ( Fig. 4 ; Supplementary Fig. 2 ; Supplementary Table 3 ). In contrast, m =0 could not be rejected for Silver-backed to Grey Butcherbirds, for Black-backed to Grey Butcherbirds and in both directions between Black-backed and Silver-backed Butcherbirds (that is, peak probabilities were close to and included zero; Fig. 4 ; Supplementary Fig. 2 ; Supplementary Table 3 ). 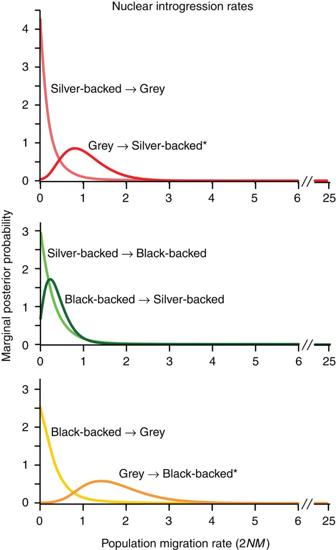Figure 4: Test of nuclear introgression between currently allopatric species. Marginal posterior probability distributions for population migration rate (2NM) estimated by IMa2 when Silver-backed and Black-backed Butcherbirds are inferred to be sister species (Tree 1). Estimates were substantially different from zero for both Grey into Silver-backed Butcherbirds and Grey into Black-backed Butcherbirds. Combined with the inferences from STRUCTURE and *BEAST, these data support species-level recognition for Grey (C. torquatus, Latham, 1802), Black-backed (C. mentalis, Salvadori & d’Albertis, 1876) and Silver-backed Butcherbirds (C. argenteus, Gould, 1841) under a species concept that allows for some low-level gene exchange between evolutionary independent lineages (for example, Phylogenetic and Evolutionary Species Concepts). Figure 4: Test of nuclear introgression between currently allopatric species. Marginal posterior probability distributions for population migration rate (2NM) estimated by IMa2 when Silver-backed and Black-backed Butcherbirds are inferred to be sister species (Tree 1). Estimates were substantially different from zero for both Grey into Silver-backed Butcherbirds and Grey into Black-backed Butcherbirds. Combined with the inferences from STRUCTURE and *BEAST, these data support species-level recognition for Grey ( C. torquatus , Latham, 1802), Black-backed ( C. mentalis , Salvadori & d’Albertis, 1876) and Silver-backed Butcherbirds ( C. argenteus , Gould, 1841) under a species concept that allows for some low-level gene exchange between evolutionary independent lineages (for example, Phylogenetic and Evolutionary Species Concepts). Full size image Tests for population size change Demographic history was inferred using the extended Bayesian skyline model, EBSP [32] in BEAST v1.7.5 (ref. 33 ) and Tajima’s D, R2 and Fu’s Fs tests for deviations from neutrality for each locus in DnaSP v5 (ref. 34 ). Grey Butcherbirds were the only species that showed significant deviations from neutrality and assumptions of constant population size (Tajima’s D, P <0.05: BF-7 ; Fu’s Fs, P <0.02: ND2, ACTB-3-3, BF-7 BRM-15 ; Supplementary Table 4 ). When analysed separately, eastern and western populations of Grey Butcherbirds also showed significant deviations from constant population size (that is, ND2, ACTB-3, ODC-6 & 7 ; Supplementary Table 4 ). EBSP of the combined mtDNA and nuclear data set showed a 10-fold population size expansion in Grey Butcherbirds ( Fig. 5 ). When analysed separately, each of the eastern and western Grey Butcherbirds showed a signal of population increase, although the pattern differed. The signal of population expansion in the western Grey Butcherbirds increased sharply around 30–25 kya, whereas there was a steady increase in population size in the eastern Grey Butcherbirds from 50 kya to present. There was no demographic change in either Silver-backed or Black-backed Butcherbirds in the past 50 ka ( Fig. 5 ). 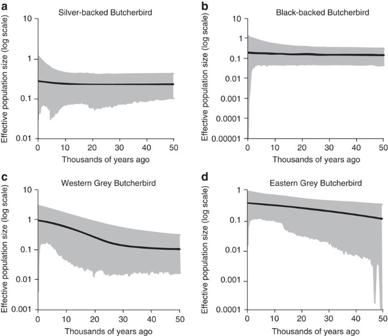Figure 5: Test of population expansion using EBSP. Extended Bayesian skyline plots estimated using combined mitochondrial and nuclear DNA sequence data of (a) Silver-backed Butcherbirds, (b) Black-backed Butcherbirds, (c) western Grey Butcherbirds and (d) eastern Grey Butcherbirds. The median posterior estimates of demographic change over the past 50,000 years are graphed with the shaded area indicating the 95% HPD. Figure 5: Test of population expansion using EBSP. Extended Bayesian skyline plots estimated using combined mitochondrial and nuclear DNA sequence data of ( a ) Silver-backed Butcherbirds, ( b ) Black-backed Butcherbirds, ( c ) western Grey Butcherbirds and ( d ) eastern Grey Butcherbirds. The median posterior estimates of demographic change over the past 50,000 years are graphed with the shaded area indicating the 95% HPD. Full size image Tests for LGM range expansion and contraction ENMs for the current interglacial and the LGM were estimated using maximum entropy species distribution modelling in MAXENT version 3.3 (ref. 35 ) from detailed species occurrence records and nine abiotic climatic variables (present-day: WorldClim database [36] ; LGM: Community Climate System Model, CCSM3 (ref. 37 )). Present-day ENMs had high area under the receiver operating characteristic curve scores (AUC: Silver-backed, 0.97; Black-backed, 0.98; Grey, 0.71; west Grey, 0.84; east Grey, 0.77; Kimberley, 0.99; Top End, 0.99) suggesting that they have good predictive power and performed significantly better than a random model (AUC: 0.5). Present-day ENMs conformed to the species range of Grey Butcherbirds and the Australian range of Black-backed Butcherbirds but predicted a broader range of suitable conditions for Silver-backed Butcherbirds (probability of occurrence >0.1) and a more limited range for Black-backed Butcherbirds in New Guinea ( Fig. 6 ). Despite the broad range of suitable conditions predicted for Silver-backed Butcherbirds, the regions with the highest predicted probability of occurrence (0.4–0.6) fell within the species range ( Fig. 6 ; Supplementary Fig. 3 ). 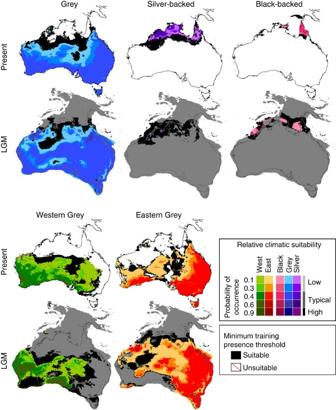Figure 6: Test of range expansions using ENM. Present day and last glacial maximum (21,000 ya) ENMs for white-throated butcherbirds. ENMs predict a northwest expansion of suitable habitats for eastern Grey Butcherbirds that could have resulted in secondary contact with Silver-backed Butcherbirds at LGM. Colours show the relative climatic suitability scores for each taxon. Regions with low suitability fall between 0.1 and 0.4 probability of occurrence, regions that are ‘typical’ of the abiotic niche of the species per taxon are 0.4–0.9, and regions that have high suitability are above 0.9 probability of occurrence. Black shows regions with suitable conditions under the less over-fit MTP threshold. Figure 6: Test of range expansions using ENM. Present day and last glacial maximum (21,000 ya) ENMs for white-throated butcherbirds. ENMs predict a northwest expansion of suitable habitats for eastern Grey Butcherbirds that could have resulted in secondary contact with Silver-backed Butcherbirds at LGM. Colours show the relative climatic suitability scores for each taxon. Regions with low suitability fall between 0.1 and 0.4 probability of occurrence, regions that are ‘typical’ of the abiotic niche of the species per taxon are 0.4–0.9, and regions that have high suitability are above 0.9 probability of occurrence. Black shows regions with suitable conditions under the less over-fit MTP threshold. Full size image ENMs predict that suitable conditions for Grey Butcherbirds expanded at LGM ( Fig. 6 ). Specifically, both the conservative minimum training presence (MTP) and the more stringent relative climatic suitability (RCS) models predict a northwest expansion of suitable conditions for eastern Grey Butcherbirds, whereas no northward expansion is predicted for western Grey Butcherbirds at LGM ( Fig. 6 ). Suitable conditions for western Grey Butcherbirds predicted under the RCS model show a contraction at LGM in south-western and central-western Australia ( Fig. 6 ). While the RCS model for Silver-backed Butcherbirds shows a considerable contraction of suitable conditions for this species at LGM ( Fig. 6 , Supplementary Fig. 3 ), the MTP model predicts a similar amount of suitable habitats to that at present ( Fig. 6 ). Suitable conditions for Black-backed Butcherbirds are predicted to have shifted west on the exposed Arafura shelf at LGM; however, there is no extensive overlap predicted between Silver-backed and Black-backed Butcherbirds ( Fig. 6 ). Our goal was to assess whether the history of the white-throated butcherbirds was shaped by range expansions or contractions during Pleistocene GM using a series of predictions for each alternative model. Multiple lines of evidence support the idea that the arid-tolerant Grey Butcherbird had a more extensive range during GM than at present. These include (1) phylogeographic and coalescent support for nuclear and mtDNA introgression of Grey Butcherbirds into Silver-backed Butcherbirds, and no introgression between Silver-backed Butcherbirds and Black-backed Butcherbirds ( Fig. 4 ), (2) ENM predictions of a substantial northwestward range expansion of Grey Butcherbirds that could have resulted in secondary contact with Silver-backed Butcherbirds at LGM ( Fig. 6 ) and (3) a 10-fold population size expansion in Grey Butcherbirds that was not seen in either Silver-backed or Black-backed Butcherbirds ( Fig. 5 ). Together, these data show that a model of GM range expansion ought to be considered for other arid-tolerant biota in Australia rather than the dominant assumption that all Australian biota contracted to GM refugia. Our data specifically fit a scenario where Silver-backed Butcherbirds are sister to Black-backed Butcherbirds, and where introgression from eastern Grey Butcherbirds led to the replacement of putatively parental Clade 2 haplotypes with Grey Butcherbird haplotypes from Clade 1 in the eastern part of the Silver-backed Butcherbird’s range ( Fig. 7a ). At this stage, coalescent modelling is insufficiently accurate to estimate the precise timing or frequency of secondary contact [38] . Thus, we cannot determine whether secondary contact between Silver-backed and eastern populations of Grey Butcherbirds occurred during, or before, the LGM. Critically, our ENMs require further validation with alternative climate models (for example, FGOALS-g1.0 and MIROC3.2—available at the Paleoclimate Modelling Intercomparison Project site, http://pmip2.lsce.ipsl.fr/ ) since these can produce different results from the CCSM3 model employed in this study. We note, however, that ENMs showing an LGM range expansion in Grey Butcherbirds ( Fig. 6 ) are concordant with independent palaeoclimatic reconstructions for Australia ( Fig. 1 ) [7] , [8] that show habitats more conducive to close contact between the savanna-inhabiting Silver-backed Butcherbird and the arid-tolerant Grey Butcherbird during arid GM rather than warmer and wetter interglacials, such as at present. Furthermore, our finding of unidirectional introgression from Grey into Silver-backed Butcherbirds is consistent with theoretical predictions that the direction of introgression should be from the higher density population to the lower [39] . Larger population sizes were estimated in Grey Butcherbirds throughout the past 50 ka than in Silver-backed Butcherbirds ( Fig. 5 ), and ENMs predicted low suitability habitats for Silver-backed Butcherbirds but high suitability habitats for eastern Grey Butcherbirds in the region of secondary contact at LGM ( Fig. 6 ). Together, this supports the idea that eastern Grey Butcherbirds invaded the habitat of Silver-backed Butcherbirds during GM. 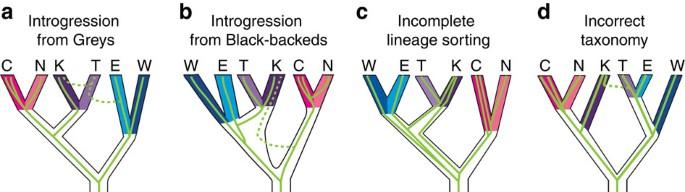Figure 7: Four alternative hypotheses to explain the origin of mtDNA paraphyly in Silver-backed Butcherbirds. (a) Introgression from eastern Grey Butcherbirds into Silver-backed Butcherbirds, (b) introgression from Black-backed Butcherbirds into Silver-backed Butcherbirds, (c) incomplete lineage sorting, and (d) incorrect taxonomy. Green lines represent the mtDNA gene tree embedded within four alternative species trees that are scaled by time. C, Cape York Peninsula (CYP); N, New Guinea (NG); K, Kimberley (KIM); T, Top End (TE); E, eastern Grey Butcherbirds; W, western Grey Butcherbirds. Figure 7: Four alternative hypotheses to explain the origin of mtDNA paraphyly in Silver-backed Butcherbirds. ( a ) Introgression from eastern Grey Butcherbirds into Silver-backed Butcherbirds, ( b ) introgression from Black-backed Butcherbirds into Silver-backed Butcherbirds, ( c ) incomplete lineage sorting, and ( d ) incorrect taxonomy. Green lines represent the mtDNA gene tree embedded within four alternative species trees that are scaled by time. C, Cape York Peninsula (CYP); N, New Guinea (NG); K, Kimberley (KIM); T, Top End (TE); E, eastern Grey Butcherbirds; W, western Grey Butcherbirds. Full size image mtDNA capture has not resulted in the complete replacement of parental Silver-backed mtDNA with introgressed Grey Butcherbird mtDNA. The persistence of Clade 2 haplotypes west of the Ord River ( Fig. 2 ) and the signal of a private Z-linked BRM-15 allele restricted to populations west of the Victoria River ( Fig. 3 ) in the Kimberley are consistent with a geographic barrier limiting intraspecific gene flow between Top End and Kimberley populations. Likely candidates are the Ord River arid intrusion separating the Kimberley and Victoria River sandstone plateaus, and the Victoria River arid intrusion separating the disjunct Kimberley and Top End populations of the Silver-backed Butcherbird sensu Ford [28] . These geographic barriers have been implicated in intraspecific divergences of other species in this region [12] , [40] , [41] . Alternatively, these phylogeographic patterns could result if insufficient time has elapsed since introgression for a range-wide sweep of mtDNA, or if intraspecific gene flow of mtDNA and Z-linked loci was more limited than that of autosomal loci in accordance with the expectations of Haldane’s rule [39] . Alternative explanations for the origin of mtDNA paraphyly appear unlikely ( Fig. 7 ). Introgression from Black-backed Butcherbirds into Silver-backed Butcherbirds ( Fig. 7b ) was not supported by IMa2 models ( Fig. 4 ) and the temporal and spatial structuring of mtDNA diversity invokes an unlikely biogeographic scenario requiring either that (1) secondary contact ‘leap-frogged’ the more geographically proximate Top End populations or (2) more recent gene flow between Top End populations and eastern Grey Butcherbirds ‘erased’ the signal of earlier introgression from Black-backed Butcherbirds in the Top End. Incomplete lineage sorting ( Fig. 7c ) can be rejected owing to nuclear coalescent models that do not exclusively fit an allopatric model of divergence ( Fig. 4 ; Supplementary Fig. 2 ). Incorrect taxonomy ( Fig. 7d ) can be rejected owing to congruence between phenotype and the nuclear species tree and STRUCTURE analyses ( Fig. 3 ), which clearly support the Top End and Kimberley populations as each other’s closest relatives to the exclusion of Black-backed and Grey Butcherbirds. Many other species from Australia’s drier habitats have phylogeographic histories that could fit models of GM expansion, range shift or, at least, the maintenance of large populations rather than contraction to isolated GM refugia. For example, large GM range or population sizes are predicted for Callitris trees in southern Australia [42] and Uperoleia toadlets [12] and Estrilid finches [13] in northern Australia, as well as several bird species with nearly continent-wide distributions [15] . These patterns have all been interpreted within the context of GM contractions, conceivably because of the refugia-centric legacy of our traditional ‘one-model-fits-all’ approach that focused on finding congruent GM refugia across all taxa. This failed paradigm led to conclusions of ‘multiple, idiosyncratic (species-specific), GM refugia’ for arid zone taxa in order to explain molecular evidence that large populations persisted throughout the Pleistocene [14] , [43] , [44] . Our data reinforce the idea that, rather than responses being ‘idiosyncratic’, different species ecologies and environmental heterogeneity produce discordant, but predictable, species responses to GM aridity [25] , [44] . mtDNA ( Fig. 2 ), palaeo-ENMs ( Fig. 6 ) and palaeoclimatic reconstructions ( Fig. 1a ) suggest climates that were largely hospitable for eastern Grey Butcherbirds and allowed their GM range expansions, whereas extreme aridity and extensive, treeless, sand-dunes in central and western Australia [7] likely caused GM range contractions in western Grey Butcherbirds and limited their northward range expansion. Similar patterns of increased population structure in western Australia and unstructured, star-shaped polytomies in eastern Australia have been documented in other widespread species [43] , [45] suggesting that their histories have been shaped by similar processes. There is also growing evidence that, in northern Australia, species with different ecologies have undergone discordant, but predictable, responses to GM aridity [25] , [26] , [40] , [44] , [46] . Weaker monsoons and increased GM aridity appear to have caused range disjunctions on either side of the Carpentarian Barrier (see Fig. 2 for location) in species of monsoonal savanna woodlands [40] , [46] and mesic rainforests and mangroves [25] but to have facilitated range expansion in the arid-tolerant Grey Butcherbird ( Fig. 6 ). Notably, despite predictions of GM range disjunctions [40] , [46] or range contractions/shifts (butcherbirds; Fig. 6 ), savanna woodland species likely do not fit a model of GM contraction to refugia, since these species appear to have maintained large effective population sizes throughout the Pleistocene. However, a shift from panmixia to multiple subdivided populations (for example, dispersed GM refugia or range disjunction) could theoretically cause an increase in effective population size ( Ne ) without a marked change in population size (abundance). This argues for the combined use of ENMs, phylogeography and multilocus coalescent estimates of demographic change ( Ne ) when evaluating the fit of alternative GM models rather than relying on a single line of evidence. The lack of consideration of the different effects that ecology can have on population history in Australia is surprising, given that such ecology-driven models exist for species from other continents whose responses likely parallel those of Australia’s drier habitats—for example, species of savanna habitats in Africa [9] , tropical Amazonia [2] , unglaciated regions in the northern hemisphere [3] and cold-adapted species (arctic and alpine habitats) in glaciated regions in the northern hemisphere [10] . Our next step ought to focus on developing a strong theoretical foundation against which ideas of species responses to GM aridity in Australia can be tested. This will require the development of explicit predictions of the genetic consequences and range dynamics under each alternative GM model and for different species ecologies [5] , as well as the development of tools that are able to differentiate between the similar demographic signatures produced under different processes (for example, expansion versus population subdivision). Testing of explicitly defined GM models within a comparative framework might reveal congruent responses among co-distributed species or those with similar ecologies that have otherwise been attributed to ‘discordant patterns resulting from idiosyncratic responses’ [16] , [44] . Molecular sampling approach All specimens used in this study were collected under the appropriate ethics and collecting permits from the relevant Australian States and Territories over a number of years by the Australian National Wildlife Collection (ANWC, CSIRO, Ecosystem Sciences, Canberra, Australia), Western Australian Museum (Perth, Australia), Museum Victoria (Melbourne, Australia) and the Australian Biological Tissue Collection (South Australian Museum, Adelaide Australia; see Supplementary Data 1 ). Specimens collected by the ANWC specifically for this project were obtained under CSIRO Ecosystem Sciences Animal Ethics Committee Permit 10-04 Systematic Avifaunal Surveys in Western Australia and the Northern Territory; CSIRO Sustainable Ecosystems Animal Ethics Committee Permit 07-04 Avifaunal Surveys of the Great Victoria Desert; CSIRO Human Nutrition Animal Ethics Committee Permit no. 713-08/08; Permits SF006336 and SF 007359 from the Western Australian Department of Environment and Conservation; Permit 37355 from the Northern Territory Department of Natural Resources, Environment, the Arts and Sport and Permit Y25496-1 from the South Australian Department for Environment and Heritage. The mitochondrial ND2 locus was sampled for 138 white-throated butcherbirds representing all named species (Silver-backed , n =36; Black-backed , n =13; Grey, n =89; Supplementary Data 1 for sample details). Seven nuclear introns ( ACTB-3 , BF-7 , FN1-31 , GAPDH-11 , ODC-6&7 , RPL37A-3 and BRM-15 ) were sampled for a subset of individuals ( Supplementary Data 1 for sample sizes at each locus). This study adds to the data set of the previously published systematic study of Kearns et al. [23] comprising five nuclear introns ( BF-7 , BRM-15 , GAPDH-11 , ODC-6 & 7 and CHDZ-18 ) and one mtDNA locus ( ND2 ) sampled for 81 white-throated butcherbirds (Silver-backed, n =32; Black-backed, n =13; Grey, n =36). CHDZ-18 was omitted from this study as it was invariable in white-throated butcherbirds. Introns ACTB-3 , FN1-31 and RPL37A-3 were sequenced specifically for this study. Cryofrozen tissue samples were available from the ranges of all three species; however, there were limited samples available for Silver-backed and Black-backed Butcherbirds, and so the study of these species relied heavily on toe-pad tissues from museum specimens. ND2 sequences from five species, including representatives from Cracticus and other Artamidae, were obtained from GenBank and included as outgroups for the mtDNA data set ( Supplementary Data 1 ). DNA amplification and sequencing Frozen tissues were digested for 24 h using proteinase K and lysis buffer, and then genomic DNA was extracted using ammonium acetate and ethanol precipitation (see Kearns et al. [26] for further details). Toe-pad samples were extracted using a DNeasy Tissue Kit (Qiagen, Valencia, CA, USA) with modifications to the manufacturer’s protocol to improve the yield for degraded samples including manually abrading the toe-pad sample to increase the surface area that is being digested, increasing the digestion time, increasing the volume of proteinase K and reducing the volume of elution buffer (see Kearns et al. [25] for further details). To minimize the risk of contamination, DNA extraction and PCR of toe-pad samples were performed in a separate laboratory that had no contact with bird tissues or PCR products. To increase the chance of detecting contamination, all samples were extracted and sequenced with toe-pad samples from other Cracticus species, DNA extraction- and PCR-negatives were sequenced, and both frozen tissue and toe-pad tissues from one C. quoyi [25] and two C. mentalis specimens were extracted and sequenced for ND2 and BRM . PCR amplification used 1.5 μl of MgCl 2 (50 μM), 5 μl of 5 × buffer, 2 μl of dNTPs (2 μM), 0.5 μl of each primer (10 μM), 0.2 μl of MangoTaq and template DNA and thermocycle conditions calibrated for tissue type and locus (see Supplementary Table 5 for details). Toe-pad samples were purified using ExoSAP. Frozen tissues were purified using ammonium acetate (7.5 M) precipitation. Sequencing was performed by Macrogen (Seoul, Korea). CodonCode Aligner 3.0.1 (CodonCode Corporation, 2002–2009) was used to edit and align sequences. PHASE v2.1 (ref. 47 ) was used to infer the gametic phase of individuals with multiple heterozygous sites from five independent runs (-x5 algorithm) with a 0.70 posterior probability threshold. The subtraction method was used to infer phase for individuals that were heterozygous for indels (length-variant heterozygotes) [48] . The four-gamete test implemented in DnaSP v5 (ref. 34 ) was used to test for recombination, and the longest independently segregating (non-recombining) block of sequence data from each locus was used in subsequent analyses. Single-locus phylogenies and networks Bayesian inference was used to estimate the mtDNA gene tree in MrBayes 3.1.2 (ref. 49 ). Two analyses were run for 10 million generations, each using codon position partitions and the GTR+I+G substitution model and with four chains, default heating values and sampling every 100,000 generations. Convergence and the appropriate burnin were determined by comparing harmonic means and trend plots from the two runs. Unrooted allele networks for the nuclear and mtDNA loci were constructed using the union of maximum parsimony trees method in the programme CombineTrees [50] using the following steps for each locus: (a) identical sequences were merged using MacClade 4.06 (ref. 51 , b) multinucleotide indels were reduced to 1 bp to take advantage of the ‘gap as fifth base’ option in PAUP* 4.0b10 (ref. 52 , c) maximum parsimony trees were estimated in PAUP* using tree-bisection-reconnection branch-swapping algorithm and simple sequence addition, (d) the maximum parsimony trees were input into CombineTrees and combined into a single reticulated network using default settings. Measures of net-sequence divergence ( Dxy ) and descriptive statistics were calculated for each locus in DnaSP v5 (ref. 34 ). The degree of population structure was investigated using analysis of molecular variance in Arlequin v3.11 (ref. 53 ; permutations=10,000; significance level=0.05). Multilocus tests of species boundaries *BEAST [32] analyses used a Yule speciation prior on the species tree and applied a strict clock for all nuclear loci after preliminary runs rejected a relaxed clock for these loci (s.d. of the substitution rate parameter included zero). The best-fit substitution model for each locus as selected in MrModeltest 2.2 (ref. 54 ) under the Akaike information criterion was used in *BEAST analyses: ACTB-3 : HKY+I, BF-7 : HKY, BRM-15 : GTR, FN1-31 : HKY, GAPDH-11 : HKY+I, ODC-6&7 : HKY, RPL37A-3 : GTR+I. *BEAST was run twice for 8 × 108 generations, sampling every 5,000 generations and with a burnin of 8 × 107 generations. Convergence was assessed using TRACER v1.5 (ref. 55 ) by ensuring that effective sample size (ESS) values were above 200 and that independent runs had converged on the same stationary distribution. LOGCOMBINER v1.6.1 (ref. 55 ) was used to combine the two runs, and then TREEANNOTATOR v1.6.1 (ref. 55 ) was used to generate a maximum-clade-credibility tree from the 288,000 post-stationarity trees. STRUCTURE [30] analyses used a subset of 51 individuals that had near complete sampling for all seven nuclear loci (see Supplementary Data 1 for sampling details). Twenty runs of one million generations with 100,000 generations discarded as burnin were performed for each value between K =1 and K =8 using the admixture model and with allele frequencies correlated among populations. STRUCTURE HARVESTER v0.6.8 (ref. 56 ) was used to implement the delta K method, which examines the rate of change in the log probabilities of each value of K in order to determine the best value of K for the data [57] . CLUMPP [58] was used to combine independent results from the 20 replicated runs for K =2, 3, 4 and 6 using the ‘Full Search’ option ( M =1) and default settings. Tests for introgression Demographic parameters (divergence time ( t ), effective population size ( Ne ) and population migration rate ( 2NM )) were estimated from the nuclear intron data set using the ‘Isolation-with-Migration-analytic model for more than two populations’ (IMa2) [31] . mtDNA data were not included in IMa2 models. Owing to ambiguity in the sequence of divergence of the white-throated butcherbirds (see Results), separate IMa2 models were run for the two most plausible species trees: ‘Tree 1 ((Silver-backed, Black-backed) Grey)’ and ‘Tree 2 ((Silver-backed, Grey) Black-backed)’. Several preliminary runs were performed with wide priors (for example, population size ( q )=30, migration rate ( m )=100, divergence time ( t )=20) in order to identify appropriate upper bounds that encompassed the posterior distribution of each parameter [59] . Preliminary runs implementing the full IMa2 model failed to converge and mix adequately, thus ‘ancestral migration’ (gene flow after t 1 and before t 0 ) was eliminated from final analyses (-j3 option) to reduce the complexity of the model. For both species trees, estimates for t and ancestral population size did not have closed posterior densities—posterior densities either (a) extended indefinitely at low probabilities (ancestral population size) or (b) peaked early, dropped and plateaued at low probabilities ( t ). Following the recommendations of Won & Hey [59] and Hey [60] , the upper bound of the prior for these two parameters was constrained to a lower, more biologically meaningful, value. Final IMa2 analyses used 80 independent Markov-coupled chains with a geometric heating scheme (g1=0.96, g2=0.5). The infinite-site mutation model was applied to each locus. After an initial run using a burnin of 2,000,000 steps and a run length of 2,000,000 steps, several independent runs (burnin=100,000–2,000,000 steps; run length=2,000,000–15,000,000 steps) were started from the Markov chain state files of previous runs using different random number seeds. For each species tree model, final demographic parameter estimates were recorded from two independent runs initiated from identical Markov chain state files with different random number seeds (Guide tree 1: 100,000 burnin, 6,000,000 run length; Guide tree 2: 100,000 burnin, 10,000,000 run length). Parameter convergence and chain mixing were assessed using the following criteria: (a) low autocorrelation of parameters (<0.1), (b) absence of discernible trends in plots for L[P] and t parameters, (c) ESSs above at least 70 (typically >100–1,000) and (d) consistency of results across replicated runs [60] . Model parameters were converted into biologically meaningful demographic parameters (that is, divergence time in years, effective population size ( Ne ) and population migration rate (2 NM )) using a generation time of two years (based on the age of first breeding of Grey Butcherbirds [61] ), a neutral mutation rate of 1.35 × 10−9 substitutions per site per year (estimated for nuclear introns for birds [62] ), and inheritance scalars of 1.0 for autosomal and 0.75 for Z-linked loci. Tests for population size change Demographic history was inferred using the extended Bayesian skyline model, EBSP [32] in BEAST v1.7.5 (ref. 33 ), and tests for deviations from neutrality and assumptions of constant population size using the Tajima’s D, Fu’s Fs and R2 statistics in DnaSP v5 (ref. 34 ) for each locus. Independent EBSP analyses partitioned by loci were run for Grey Butcherbirds, Silver-backed Butcherbirds and Black-backed Butcherbirds. The Bayesian skyline model assumes sampling from a panmictic population and sampling from structured populations can lead to false inferences of population decline [63] . To account for potential problems arising from mtDNA structure identified for Grey Butcherbirds, we also ran EBSP separately for eastern and western populations of Grey Butcherbirds. For each locus partition, evolutionary models were selected using MrModeltest [54] (see Supplementary Table 6 ). We selected a strict clock for each analysis based on population-level structure within each species. Analyses were run starting with a random tree. We specified a substitution rate of 2.9 × 10 −2 substitutions per site per million years [64] for ND2 and estimated substitution rates for all nuclear loci. A normal prior was selected for the ND2 substitution rate with a s.d. of 0.003, which was estimated from the 95% HPD (2.4–3.3 × 10 −2 substitutions per site per million years) in Lerner et al. [64] For all other loci, we selected a gamma prior distribution (shape 1.0, scale 0.01) on the clock rate to reflect prior knowledge of a slower rate for the nuclear loci than ND2 . BEAST runs were sampled every 2,000 generations for a total of 100 million generations to ensure effective sample size (ESS) posterior parameter estimates were greater than 100 and that stationarity of parameters was reached within the default EBSP burnin of 10%. Tests for LGM range expansion or contraction Present-day ENMs were estimated using maximum entropy species distribution modelling in MAXENT version 3.3 (ref. 35 ) from nine abiotic climatic variables (2.5-min resolution) from the WorldClim database [36] and georeferenced occurrence records (see Fig. 1b ) from the Birds Australia Birdata Project ( www.birdata.com.au ) accessed through the Atlas of Living Australia website ( www.ala.org.au ) and the Australian National Wildlife Collection (429 records of Silver-backed, 618 records of Black-backed Butcherbirds and 24,295 records of Greys (18,595 records from the east and 5,700 from the west)). Occurrence records were verified and refined according to species ranges in Schodde and Mason [22] . To avoid overfitting the model, ENMtools [65] was used to remove occurrence records within one-grid cell of each other, and to test for strong correlations among bioclimatic variables (Pearson’s correlation: R >0.90). This resulted in a final data set of nine bioclimatic variables without strong correlations ( R <0.90): Annual Mean Temperature (Bio1), Temperature Seasonality (Bio4), Mean Temperature of Wettest Quarter (Bio8), Mean Temperature of Driest Quarter (Bio9), Mean Temperature of Warmest Quarter (Bio10), Precipitation Seasonality (coefficient of variation) (Bio15), Precipitation of Wettest Quarter (Bio16), Precipitation of Warmest Quarter (Bio18) and Precipitation of Coldest Quarter (Bio19). ENMs were generated using the recommended default settings: regularization=1, iterations=500, convergence threshold=0.00001 (ref. 35 ). The accuracy of the present-day ENMs (continuous RCS models) were evaluated using the AUC (random test percentage=25%, threshold=0.70) and by visually assessing the fit of ENMs to published range limits of each species [66] . LGM ENMs were obtained by projecting present-day ENMs on bioclimatic variables predicted for the LGM under the Community Climate System Model and with ‘fade-by-clamping’ [67] . RCS predictions were converted into binary distributions depicting ‘suitable’ and ‘unsuitable’ conditions using the MTP threshold (lowest presence threshold) to provide a less over-fit interpretation of suitable climatic conditions [67] . Accession Codes: ND2 and intron sequences have been deposited in GenBank nucleotide database under the accession codes KC533176 to KC533433 and KC545224 to KC545225 . How to cite this article: Kearns, A. M. et al. Australia’s arid-adapted butcherbirds experienced range expansions during Pleistocene glacial maxima. Nat. Commun. 5:3994 doi: 10.1038/ncomms4994 (2014).